Recognition of vitamin B metabolites by mucosal-associated invariant T cells The mucosal-associated invariant T-cell antigen receptor (MAIT TCR) recognizes MR1 presenting vitamin B metabolites. Here we describe the structures of a human MAIT TCR in complex with human MR1 presenting a non-stimulatory ligand derived from folic acid and an agonist ligand derived from a riboflavin metabolite. For both vitamin B antigens, the MAIT TCR docks in a conserved manner above MR1, thus acting as an innate-like pattern recognition receptor. The invariant MAIT TCR α-chain usage is attributable to MR1-mediated interactions that prise open the MR1 cleft to allow contact with the vitamin B metabolite. Although the non-stimulatory antigen does not contact the MAIT TCR, the stimulatory antigen does. This results in a higher affinity of the MAIT TCR for a stimulatory antigen in comparison with a non-stimulatory antigen. We formally demonstrate a structural basis for MAIT TCR recognition of vitamin B metabolites, while illuminating how TCRs recognize microbial metabolic signatures. The αβ T-cell receptor (TCR) binds peptide and lipid-based antigens presented by the major histocompatibility complex (MHC) and CD1 families, respectively. In addition, some TCRs can recognize small organic compounds presented by MHC-like molecules, although the basis of this interaction is unknown. Mucosal-associated invariant T (MAIT) cells are an abundant population of innate-like T cells in humans that reside in the peripheral blood, but are predominantly found in the gastrointestinal mucosa and liver [1] , [2] . Although the physiological role of MAIT cells is emerging, it is established that numerous bacteria and yeast activate MAIT cells [3] , [4] , [5] , [6] . MAIT cells also require the gut microbiota for their development, and are implicated in protective immunity and several disorders caused by aberrant immunity [3] , [4] , [7] , [8] , [9] , [10] , [11] , [12] . MAIT cells, like type I natural killer T-cells (NKT cells), rapidly secrete a range of cytokines upon activation through a receptor selected from the adaptive αβ TCR repertoire that is expressed on their cell surface [5] . The NKT TCR specifically recognizes a variety of synthetic, self and foreign lipid-based ligands bound to CD1d [13] , [14] , whereas the MAIT TCR is restricted to the ubiquitously expressed MHC-I-related molecule [15] , MR1, which presents vitamin B-based metabolites to MAIT cells [16] . Consistent with their innate-like phenotype, MAIT and NKT cells express a very restricted T-cell repertoire, in contrast to the enormously diverse T-cell repertoire often observed in MHC-restricted immunity [17] , [18] , [19] . Human MAIT cells are characterized by an invariant TCR α-chain (TRAV1–2–TRAJ33) paired with a limited array of TCR β-chains (TRBV6 or TRBV20) [17] , whereas human type I NKT cells express an invariant α-chain (TRAV10–TRAJ18) coupled to a TRBV25-1-encoded TCR β-chain [20] . A high level of conservation of MR1 in mammals, and the restricted MAIT TCR usage, strongly indicates an important and evolutionarily conserved function for the MAIT TCR–MR1 axis in immunity [21] . We recently described a family of vitamin B-related ligands presented by MR1 that exhibit variable potency for MAIT cells [16] . Central to understanding the MAIT cell function is the basis for the highly restricted MAIT TCR α-chain selection, the nature of the MAIT TCR–MR1–Ag interaction, the mechanisms by which the MAIT TCR discriminates between MR1-bound vitamin B metabolites, and the basis of MAIT cell agonism. Here we present the crystal structures of the MAIT TCR bound to MR1 presenting a non-agonist and an agonist antigen. We provide insight into the invariant MAIT TCR α-chain usage, MR1 restriction and, importantly, provide definitive insight into TCR recognition of vitamin B metabolites, thereby providing the molecular basis for MAIT cell agonism. Overview of the MAIT TCR–MR1–Ag complex Although a folic acid metabolite (6-formyl pterin, 6-FP) did not activate MAIT cells, riboflavin derivatives, including 7-hydroxy-6-methyl-8-D-ribityllumazine (RL-6-Me-7-OH), specifically stimulated MAIT cells in an MR1-restricted manner [16] . Although the MR1-restricted ligands, including 6,7-dimethyl-8-D-ribityllumazine and reduced 6-hydroxymethyl-8-D-ribityllumazine, refolded very inefficiently with MR1 (thereby hampering structural studies), 6-FP and RL-6-Me-7-OH refolded sufficiently well with MR1 to enable structural studies to readily proceed. Accordingly, to definitively establish how a MAIT TCR binds stimulatory and non-stimulatory MR1–antigen complexes, we expressed and refolded a MAIT TCR (TRAV1–2–TRAJ33–TRBV6-1) (not shown) and crystallized it in complex with MR1-6-FP and MR1–RL-6-Me-7-OH. 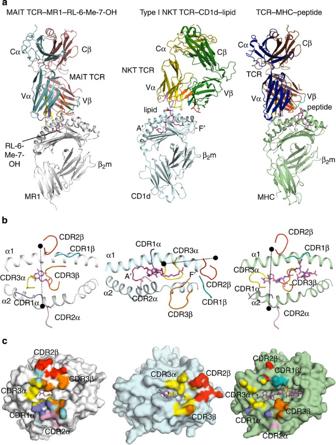Figure 1: Docking mode of the MAIT TCR in comparison with an NKT TCR that binds CD1d–lipid and a conventional TCR that binds MHC-I–peptide. (a) Left, MAIT TCR in complex with MR1–RL-6-Me-7-OH. MAIT TCR α-chain, cyan; MAIT TCR β-chain, salmon; CDR1α, purple; CDR2α, pink, CDR3α, yellow; CDR1β, teal; CDR2β, red; CDR3β, orange; RL-6-Me-7-OH, magenta; and MR1, grey. Middle, type I NKT TCR in complex with CD1d-lipid. NKT TCR α-chain, yellow; NKT TCR β-chain, green; lipid, magenta; CD1d, pale cyan; CDR loops colour coding as ina. Right, conventional TRAV1–2 TCR in complex with an MHC-peptide TCR α-chain, blue; TCR β-chain, brown; MHC, pale green; peptide, magenta; CDR loops colour coding as ina. (b) Left, MAIT TCR–MR1–RL-6-Me-7-OH complex; middle, NKT TCR–CD1d–lipid complex; and right, conventional TRAV1–2 TCR–MHC–peptide complex viewed down into the antigen-binding cleft. Black-filled circles indicate the centre of mass for the Vα and Vβ domains; CDR loops colour coding as ina. (c) Left, footprint of the MAIT TCR on the surface of MR1–RL-6-Me-7-OH; middle, footprint of the NKT TCR on the surface of CD1d–lipid; and right, footprint of the TRAV1–2 TCR on the surface of MHC–peptide. CDR loops colour coding as ina. Both MAIT TCR–MR1–Ag ternary complexes were solved to a very high resolution ( Table 1 ), and the electron density for the vitamin B metabolites within the MR1 clefts and that at the MAIT TCR–MR1–Ag interfaces were unambiguous ( Supplementary Fig. S1 ). Apart from ligand-specific interactions (discussed below), the two MAIT TCR–MR1–Ag complexes are virtually identical. To provide a context for how TCRs can recognize vitamin B metabolites, peptides and lipids, we compared the MAIT TCR–MR1–RL-6-Me-7-OH complex with a representative TCR–MHC-I-peptide and a type I NKT TCR-CD1d-α-galactosylceramide (α-GalCer) complex ( Fig. 1a ) [22] , [23] . Table 1 Data collection and refinement statistics. Full size table Figure 1: Docking mode of the MAIT TCR in comparison with an NKT TCR that binds CD1d–lipid and a conventional TCR that binds MHC-I–peptide. ( a ) Left, MAIT TCR in complex with MR1–RL-6-Me-7-OH. MAIT TCR α-chain, cyan; MAIT TCR β-chain, salmon; CDR1α, purple; CDR2α, pink, CDR3α, yellow; CDR1β, teal; CDR2β, red; CDR3β, orange; RL-6-Me-7-OH, magenta; and MR1, grey. Middle, type I NKT TCR in complex with CD1d-lipid. NKT TCR α-chain, yellow; NKT TCR β-chain, green; lipid, magenta; CD1d, pale cyan; CDR loops colour coding as in a . Right, conventional TRAV1–2 TCR in complex with an MHC-peptide TCR α-chain, blue; TCR β-chain, brown; MHC, pale green; peptide, magenta; CDR loops colour coding as in a . ( b ) Left, MAIT TCR–MR1–RL-6-Me-7-OH complex; middle, NKT TCR–CD1d–lipid complex; and right, conventional TRAV1–2 TCR–MHC–peptide complex viewed down into the antigen-binding cleft. Black-filled circles indicate the centre of mass for the Vα and Vβ domains; CDR loops colour coding as in a . ( c ) Left, footprint of the MAIT TCR on the surface of MR1–RL-6-Me-7-OH; middle, footprint of the NKT TCR on the surface of CD1d–lipid; and right, footprint of the TRAV1–2 TCR on the surface of MHC–peptide. CDR loops colour coding as in a . Full size image The MAIT TCR docked approximately centrally and orthogonally to the main axis of the MR1–Ag-binding cleft, interacting with residues spanning 61–72 and 148–164 of the α1 and α2 helices of MR1, respectively ( Fig. 1a ). The MAIT TCR–MR1–Ag docking topology starkly contrasted with the consensus type I NKT TCR–CD1d–lipid interaction, whereupon the NKT TCR docked parallel to and above the F′-pocket of the CD1d–antigen complex ( Fig. 1a–c ) [13] . Although TCRs can engage the MHC peptide in a range of docking modes [24] , the MAIT TCR–MR1–Ag complex was analogous to typical TCR–MHC-I–peptide docking, in which the α and β chains of the MAIT TCR were positioned over the α2 and α1 helices of MR1, respectively ( Fig. 1a ). Indeed, there was similarity in the overall docking mode between a TRAV1–2 TCR–HLA-B*35:01–peptide complex [22] and the MAIT TCR–MR1–RL-6-Me-7-OH complex. This similarity was surprising, given that the Vβ8.2 + TCRs adopt markedly different footprints on MHC and CD1d [25] . Further, the respective interatomic contacts differed markedly, which is partly due to a lack of sequence identity between MR1 and MHC-I at the site of the MAIT TCR footprint ( Fig. 1c , Supplementary Fig. S2 ). Moreover, there was little sequence identity between MR1 and the CD1 family at this interaction site, suggesting that there will be little in common between how TCRs can engage CD1 and MR1 ( Supplementary Fig. S2 ). The buried surface area (BSA) at the MAIT TCR–MR1–Ag interface was approximately 1,200 Å 2 , which falls within the upper end of the range of BSA values for TCR–MHC-I–peptide interactions (600–1,200 Å 2 ) and outside the range of NKT TCR–CD1d–lipid interactions (760–910 Å 2 ) [13] , [24] , [26] . However, RL-6-Me-7-OH contributed merely 0.6% of the BSA at the MAIT TCR–MR1–RL-6-Me-7-OH interface, whereas the 6-FP ligand did not contribute at all. This low % BSA contribution from the MAIT agonist ligand contrasts with the range that peptides contribute to the TCR–MHC-I–peptide interface (10–25% BSA), and is more analogous to how only a small component of lipid Ags are directly available for NKT TCR contact [13] , [24] . Thus, MR1 dominates the interactions with the MAIT TCR ( Supplementary Tables S1 and S2 ), which was characterized mostly by hydrophobic contacts. Basis of MAIT TCR β-gene usage The α- and β-chain of the MAIT TCR contributed almost equally to the BSA at the MAIT TCR–MR1–Ag interface. The MAIT TCR β-chain is biased towards TRBV6-1, TRBV6-4 and TRBV20 usage [17] . Although the CDR1β loop did not contact MR1–Ag, the CDR2β loop abuts the α1 helix, and makes 13% BSA upon complexation ( Fig. 1c ). There are a large number of polar residues at the CDR2β–MR1 contact zone, but only one CDR2β residue (Thr54β) H-bonds to MR1, and thus van der Waals contacts underpin the CDR2β–MR1 interaction ( Fig. 2a ). Nevertheless, three neighbouring framework residues (Tyr48β, Thr55β and Asp56β) that flank the CDR2β loop also add to the TCR β-chain–MR1 interface (8.4% BSA) ( Fig. 1c ), which includes a H-bond between Tyr48β OH and Arg61 from MR1 ( Fig. 2a ). Mostly, the Vβ-mediated interactions seem non-ideally disposed to interact with MR1, consistent with previous mutagenesis studies on the TRBV20–MAIT TCR, which suggested that no individual Vβ residue is essential for MAIT cell activation [27] . Further, there is no sequence identity in the corresponding CDR1β and 2β loops between the TRBV6-1/6-4 and TRBV20 genes [27] . This suggests that the Vβ bias in the MAIT TCR usage may be attributable to preferential pairing with the MAIT TCR α-chain to generate MR1-restricted TCRs. 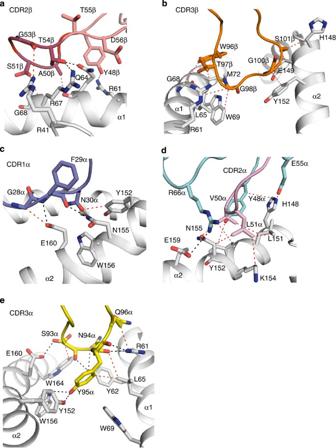Figure 2: Contacts between MAIT TCR and MR1–RL-6-Me-7-OH. (a) Contacts between CDR2β and CDR2β framework residues and MR1. (b) Contacts between CDR3β and MR1. (c) Contacts between CDR1α and MR1. (d) Contacts between CDR2α and TCRα chain framework residues and MR1. (e) Contacts between CDR3α and MR1. MR1, grey; CDR2β, red; CDR2β framework, salmon; CDR3β, orange; CDR1α, purple; CDR2α, pink; TCRα chain framework, cyan; and CDR3α, yellow. H-bond and van der Waals interactions are shown in black- and red-dashed lines, respectively. Figure 2: Contacts between MAIT TCR and MR1–RL-6-Me-7-OH. ( a ) Contacts between CDR2β and CDR2β framework residues and MR1. ( b ) Contacts between CDR3β and MR1. ( c ) Contacts between CDR1α and MR1. ( d ) Contacts between CDR2α and TCRα chain framework residues and MR1. ( e ) Contacts between CDR3α and MR1. MR1, grey; CDR2β, red; CDR2β framework, salmon; CDR3β, orange; CDR1α, purple; CDR2α, pink; TCRα chain framework, cyan; and CDR3α, yellow. H-bond and van der Waals interactions are shown in black- and red-dashed lines, respectively. Full size image Surprisingly, the majority of the TCR β-chain interactions (24.6% BSA) arose from the non-germline-encoded CDR3β loop, which, although proximal to the bound Ag, exclusively contacted MR1 directly ( Fig. 1c ). The CDR3β–MR1 interactions were chiefly hydrophobic in nature ( Supplementary Tables S1 and S2 ). Although interactions via Gly100β and Ser101β contributed to the CDR3β–MR1 interface, a ‘ 96 Trp–Thr–Gly 98 ’ sequence had a dominant role in the CDR3β-mediated contacts. Trp96β lies flat against the α1 helix of MR1, packing against Gly68 and Met72, whereas Thr97β and Gly98β form hydrophobic interactions with Arg61, Leu65 and Trp69, with Leu65 having been previously implicated as an important contact residue ( Fig. 2b ) [27] . The diverse nature of the CDR3β loop in the MAIT TCR repertoire [17] , and its location within the MAIT TCR–MR1–Ag complex, indicates that CDR3β variability may have a direct impact on the extent of self-reactivity with MR1–antigen. Basis of MAIT TCR invariant gene usage MAIT cells are characterized by germline-encoded invariant TCR α-chain usage (TRAV1–2–TRAJ33), with a variable residue encoded at the V–J junction, which does not contact MR1–Ag (not shown). The CDR1α, CDR2α, Vα framework region and the CDR3α loops contributed 6.8, 11.0, 12.0 and 22% to the BSA of the MAIT TCR–MR1–Ag interface, respectively ( Fig. 1c ). Accordingly, the CDR3α loop of the MAIT TCR α-chain made the greatest contribution to the interface, consistent with the selection of the invariant TRAJ33 gene segment in MAIT cells ( Fig. 1c ). The Gly28α–Phe29α–Asn30α cluster of residues ( Fig. 2c ), which help fix the CDR1α loop to MR1, are encoded exclusively by the TRAV1 gene family. Moreover, Phe29α is totally conserved across all mammalian TRAV1–2 orthologues ( Supplementary Fig. S3 ), highlighting the functional role of this residue in MAIT–MR1 co-evolution. The CDR2α loop resides at the periphery of the interface ( Fig. 1b ), with two ‘hydrophobic pegs’ (Val50α and Leu51α) sitting in an MR1 ‘notch’ that is lined by Leu151 and Tyr152, and the aliphatic moieties of Lys154 and Asn155 ( Fig. 2d ). Interestingly, the Leu151Ala mutant can moderately increase MAIT TCR autoreactivity [21] , [27] , thereby further highlighting the role of this MR1 residue in MAIT TCR recognition. Flanking the ‘hydrophobic peg’ are two Vα-encoded framework residues, Tyr48α and Arg66α, which collectively form a series of interactions with MR1 ( Fig. 2d ). Tyr48α packs against His148 and points towards Tyr152, whereas Arg66α salt bridges to Glu159 and H-bonds with Asn155 ( Fig. 2d ). Evolutionarily, these CDR2α-framework positions are either totally conserved across mammalian TRAV1–2 orthologues or exhibit synonymous substitutions ( Supplementary Fig. S3 ). The TRAJ33-encoded CDR3α loop sits between the helical jaws of the MR1 cleft, having a principal role in contacting both the α1 and α2 helices of MR1 and the antigen itself (discussed below) ( Supplementary Tables S1 and S2 ). Three residues at the tip of the CDR3α loop (Ser93α, Asn94α, Tyr95α) engage MR1 and this particular germline configuration is not present in any of the other 60 TRAJ genes ( Fig. 2e ). Three TRAJ33-encoded residues have a prominent role in the interaction: Ser93α H-bonds to Glu160, and its backbone H-bonds to Tyr62 OH ; Asn94α backbone packs against and H-bonds to Arg61. Tyr95α acts as a lynch-pin, in that it protrudes deep into the MR1–Ag-binding cleft, with its hydroxyl group H-bonding to Tyr152 OH , while its aromatic ring is surrounded by a nest of aromatic residues that includes Tyr62, Trp69, Tyr152 and Trp156 ( Fig. 2e ). Accordingly, Tyr95α represents a principal player in the invariant TRAJ33 use of the MAIT TCR. Of note, Tyr95α is totally conserved across all known mammalian TRAJ33 orthologues. Collectively, only TRAV1–2–TRAJ33 and none of the other 102 variable or joining genes in the human TCR α-locus encode the correct architecture required to maintain archetypal docking to MR1. In addition, key anchor sites within these receptor genes (Asn30α, Tyr48α, Val50α, Leu51α and Arg66α, Ser93α, Asn94α, Tyr95α and Gln96α) are highly conserved across eutherian and marsupial mammal orthologues, which suggest that the mode of MAIT TCR–MR1 recognition has remained relatively unchanged for 150–180 million years [28] . MR1 plasticity upon MAIT TCR binding In addition to determining the nature of the TCR contacts with the vitamin B metabolites, a comparison of the non-liganded TRAV1–2–TRAJ33–TRBV20 MAIT TCR structure and the binary MR1-6-FP complex [16] , [27] allowed us to simultaneously address the extent of conformational change within the MAIT TCR α-chain and MR1–6-FP upon ligation. Within the binary MR1–6-FP complex, the 6-FP moiety was sequestered closely within the MR1 cleft, such that 6-FP was virtually inaccessible for direct MAIT TCR contact ( Fig. 3a ) [16] . Interestingly, while the MAIT TCR α-chain and the 6-FP ligand itself did not move upon MAIT TCR–MR1–6-FP ligation, the MR1–Ag-binding cleft was more malleable ( Fig. 3b ). To accommodate the incoming Tyr95α residue from the CDR3α loop and the neighbouring CDR3β loop, a region of the α2-helix (144–153) of MR1 was ‘prised open’ upon MAIT TCR engagement ( Fig. 3b ). This prising apart of the MR1 cleft, and the displacement of Tyr152, resulted in greater solvent exposure of 6-FP ( Fig. 3c ). Nevertheless, there was no direct contact between the MAIT TCR and 6-FP in the ternary complex, although Tyr95α OH formed a water-mediated H-bond with the N1 atom of 6-FP ( Fig. 4a ). Notably, the lack of direct MAIT TCR–6-FP contacts was consistent with 6-FP being a non-stimulatory antigen and the very low affinity of this interaction ( K D(eq) >300 μM). Of note, 6-FP is a competitive inhibitor of MAIT activation as it reduces RL-6-Me-7-OH and rRL-6-CH 2 OH-induced activation of Jurkat cells transduced with three distinct MAIT TCRs in a dose-dependent manner ( Fig. 5 ). 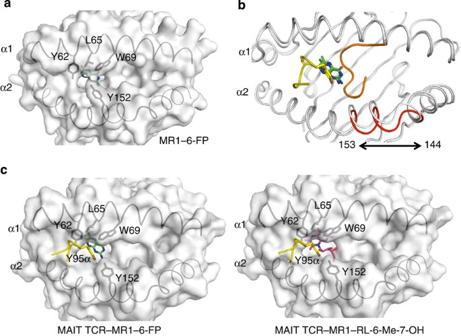Figure 3: Conformational flexibility of the MR1–antigen-binding cleft. (a) Antigen-binding cleft of MR1 with 6-FP bound. The surface is transparent to show 6-FP. (b) Cartoon overlay of the antigen-binding clefts of MR1–6-FP and MAIT TCR–MR1–6-FP. Movement of the MR1 α2 helix region 144–153 upon MAIT TCR binding is shown in red. (c) Left, antigen-binding cleft of MR1 within the MAIT TCR–MR1–6-FP complex. Right, antigen-binding cleft of MR1 within the MAIT TCR–MR1–RL-6-Me-7-OH complex. The surface is transparent. MR1, grey; 6-FP in MR1–6-FP, dark green; 6-FP in MAIT TCR–MR1–6-FP complex, green; RL-6-Me-7-OH, magenta; CDR3α, yellow. Figure 3: Conformational flexibility of the MR1–antigen-binding cleft. ( a ) Antigen-binding cleft of MR1 with 6-FP bound. The surface is transparent to show 6-FP. ( b ) Cartoon overlay of the antigen-binding clefts of MR1–6-FP and MAIT TCR–MR1–6-FP. Movement of the MR1 α2 helix region 144–153 upon MAIT TCR binding is shown in red. ( c ) Left, antigen-binding cleft of MR1 within the MAIT TCR–MR1–6-FP complex. Right, antigen-binding cleft of MR1 within the MAIT TCR–MR1–RL-6-Me-7-OH complex. The surface is transparent. MR1, grey; 6-FP in MR1–6-FP, dark green; 6-FP in MAIT TCR–MR1–6-FP complex, green; RL-6-Me-7-OH, magenta; CDR3α, yellow. 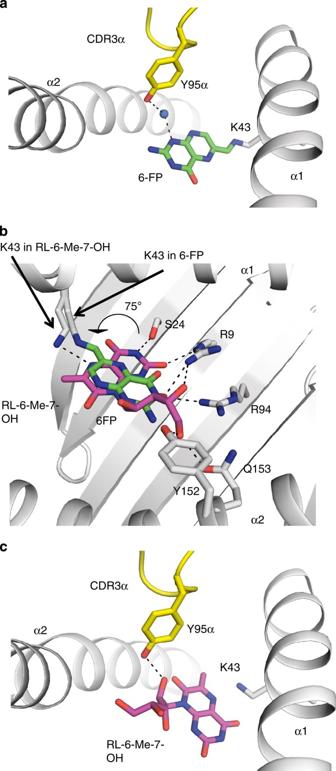Figure 4: Differences between MAIT TCR–MR1–6-FP and MAIT TCR–MR1–RL-6-Me-7-OH complexes. (a) Water-mediated interaction between CDR3α of MAIT TCR and 6-FP. (b) Overlay of MAIT TCR–MR1–6-FP and MAIT TCR–MR1–RL-6-Me-7-OH complexes. Arrow indicates 75° rotation of RL-6-Me-7-OH compared with 6-FP. (c) H-bond interaction between CDR3α of MAIT TCR and RL-6-Me-7-OH. MR1, grey; CDR3α, yellow; 6-FP, green; RL-6-Me-7-OH, magenta; blue circle, water molecule; H-bond interactions are shown in black dashed lines. Full size image Figure 4: Differences between MAIT TCR–MR1–6-FP and MAIT TCR–MR1–RL-6-Me-7-OH complexes. ( a ) Water-mediated interaction between CDR3α of MAIT TCR and 6-FP. ( b ) Overlay of MAIT TCR–MR1–6-FP and MAIT TCR–MR1–RL-6-Me-7-OH complexes. Arrow indicates 75° rotation of RL-6-Me-7-OH compared with 6-FP. ( c ) H-bond interaction between CDR3α of MAIT TCR and RL-6-Me-7-OH. MR1, grey; CDR3α, yellow; 6-FP, green; RL-6-Me-7-OH, magenta; blue circle, water molecule; H-bond interactions are shown in black dashed lines. 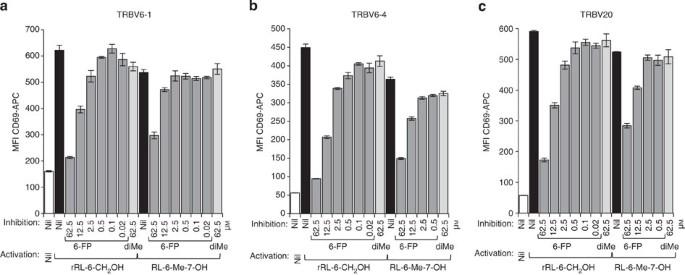Figure 5: MAIT TCR inhibition by 6-FP. C1R cells expressing human MR1 were incubated together with Jurkat.MAIT cells (105each) expressing (a) TRBV6-1, (b) TRBV6-4 or (c) TRBV20 TCRs and 6-FP or a control, pterin 6,7-dimethylpterin (di-Me), for 30 min prior to addition of RL-6-Me-7-OH or rRL-6-CH2OH, and incubation overnight. Mean fluorescence intensity of CD69 expression for gated-Jurkat.MAIT cells. Mean±s.e.m. of triplicate samples. Full size image Figure 5: MAIT TCR inhibition by 6-FP. C1R cells expressing human MR1 were incubated together with Jurkat.MAIT cells (10 5 each) expressing ( a ) TRBV6-1, ( b ) TRBV6-4 or ( c ) TRBV20 TCRs and 6-FP or a control, pterin 6,7-dimethylpterin (di-Me), for 30 min prior to addition of RL-6-Me-7-OH or rRL-6-CH 2 OH, and incubation overnight. Mean fluorescence intensity of CD69 expression for gated-Jurkat.MAIT cells. Mean±s.e.m. of triplicate samples. Full size image Interaction with vitamin B metabolites The overall features of the MAIT TCR–MR1–6FP and MAIT TCR–MR1–RL-6-Me-7-OH complexes were very similar to each other, including the more open MR1–Ag-binding cleft that increased the solvent accessibility of RL-6-Me-7-OH ( Fig. 3c , right panel). However, key differences between the complexes included the MR1–6-FP contacts differing from those of MR1–RL-6-Me-7-OH, and RL-6-Me-7-OH directly contacting the MAIT TCR. First, while 6-FP formed a Schiff base with Lys43 ( Fig. 4a ), RL-6-Me-7-OH was non-covalently bound within MR1, which resulted in Lys43 drifting away from the ligand ( Fig. 4b ). Second, and surprisingly, the orientation of RL-6-Me-7-OH within the aromatic cradle of MR1 differed dramatically from that of 6-FP. Namely, RL-6-Me-7-OH is rotated ~75° with respect to 6-FP, such that the MR1-mediated contacts between the respective ring systems differ between 6-FP and RL-6-Me-7-OH ( Fig. 4b ). The tilted conformation causes the ribityl moiety of RL-6-Me-7-OH to lean towards, and form a series of H-bonds with, Arg9 and Arg94, two evolutionarily conserved residues found within MR1 (ref. 16 ). These two Arg residues act as a platform to present the ribityl moiety in a fixed conformation to enable a direct H-bond with Tyr95α OH from the CDR3α loop of the MAIT TCR ( Fig. 4c ). Although the Tyr95α OH -mediated interaction represented the sole direct contact between the MAIT TCR and the stimulatory ligand, it nevertheless was associated with an increased affinity of interaction ( K D(eq) =1.65±0.16 μM Fig. 6a ). The importance of this Ag-centric interaction was evident from the impact of the Tyr95αPhe mutation, which markedly reduced the affinity ( K D(eq) =33.89±2.22 μM) towards the potent ligand rRL-6-CH 2 OH, as judged by SPR and cell-based activation assays ( Fig. 6b ). Thus, the principles differentiating non-stimulatory antagonist ligands and stimulatory MAIT cell antigens can be attributed to a single H-bond to the ligand itself. 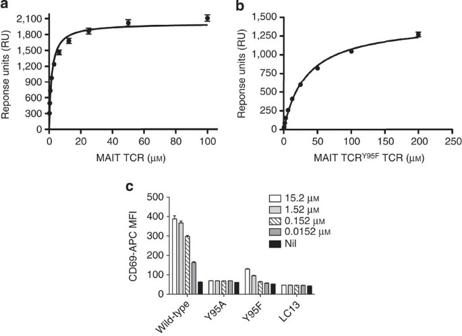Figure 6: MAIT TCR affinity for MR1 bound to antigens. SPR affinity-based measurements (at 25 °C) of the MAIT TCR binding to a potent agonist, rRL-6-CH2OH. Saturation binding curves as determined by SPR for wild-type MAIT TCR (a) or MAIT TCRY95FTCR (b). Data are representative of two independent experiments with error bars representing s.e.m. of the duplicates. (c) Activation of SKW-MAIT-TRBV6-1 cells with rRL-6-CH2OH. SKW cells transduced with genes encoding a MAIT TCR expressing wild-type or mutants Y95A, or Y95F invariant TCR α-chain (TRAV1–2–TRAJ33) paired with a TRBV6-1 β-chain were co-incubated with C1R antigen-presenting cells to which nil, or 15.2, 1.52, 0.152 or 0.0152 μM rRL-6-CH2OH was added. After 18 h SKW cells were stained and analysed by flow cytometry for cell-surface expression of CD69. Shown is the mean fluorescence intensity of staining of CD69-APC on the Y-axis. Control SKW cells expressing the EBV-specific αβ TCR LC13 (ref.40) were not activated by rRL-6-CH2OH. Data are representative of two independent experiments with error bars representing the s.e.m. of triplicate samples. Figure 6: MAIT TCR affinity for MR1 bound to antigens. SPR affinity-based measurements (at 25 °C) of the MAIT TCR binding to a potent agonist, rRL-6-CH 2 OH. Saturation binding curves as determined by SPR for wild-type MAIT TCR ( a ) or MAIT TCR Y95F TCR ( b ). Data are representative of two independent experiments with error bars representing s.e.m. of the duplicates. ( c ) Activation of SKW-MAIT-TRBV6-1 cells with rRL-6-CH 2 OH. SKW cells transduced with genes encoding a MAIT TCR expressing wild-type or mutants Y95A, or Y95F invariant TCR α-chain (TRAV1–2–TRAJ33) paired with a TRBV6-1 β-chain were co-incubated with C1R antigen-presenting cells to which nil, or 15.2, 1.52, 0.152 or 0.0152 μM rRL-6-CH 2 OH was added. After 18 h SKW cells were stained and analysed by flow cytometry for cell-surface expression of CD69. Shown is the mean fluorescence intensity of staining of CD69-APC on the Y-axis. Control SKW cells expressing the EBV-specific αβ TCR LC13 (ref. 40 ) were not activated by rRL-6-CH 2 OH. Data are representative of two independent experiments with error bars representing the s.e.m. of triplicate samples. Full size image Understanding how the immune system of the human mucosa interacts with the microbial products of the commensal microbiota and invading pathogens represents a key emerging area. We describe the molecular basis of how the immune system recognizes microbial metabolic products. Although the basis for interactions between TCRs and MHC–peptide or CD1–lipid complexes is established [25] , molecular insights into the newly discovered capacity of TCRs to interact with small organic molecules presented by MHC-like molecules is lacking. Our findings formally detail how a TCR recognizes vitamin B metabolites and, more broadly, TCR ligation to small organic metabolites bound by an Ag-presenting molecule. MAIT TCR–MR1–antigen recognition shares a mixture of key features associated with innate-like and adaptive TCR recognition [13] , [24] . Namely, the overall MAIT TCR–MR1–Ag docking topology was more similar to that of typical TCR–peptide–MHC complexes and a Type II NKT TCR–CD1d–sulfatide complex [29] , [30] . Nevertheless, the germline-encoded region of the rigid MAIT TCR contacted the minimally exposed vitamin B antigen and remoulded the MR1–Ag-binding cleft upon ligation; these features are more typical of the innate-style interactions and indicate that the MAIT TCR is an innate-like pattern recognition receptor targeted towards vitamin B metabolites. For example, the invariant NKT TCR was shown to mould the CD1d–antigen-binding cleft and deform β-linked ligands upon complexation [31] , [32] . A molecular basis for the invariant α-chain usage of the MAIT TCR is presented, showing that only a single residue within the TRAJ33 region contacts the vitamin-B-derived antigen. Thus, the principles differentiating non-stimulatory ligands and stimulatory MAIT cell antigens were attributable to a single H-bond to the ligand itself. Accordingly, understanding the molecular basis of human MAIT TCR–MR1–antigen recognition and the general principles underscoring MAIT cell agonism provides key insight into how an evolutionarily conserved and abundant innate-like T-cell population can sense microbe-derived vitamin B metabolites. MR1 and TCR preparation Genes encoding soluble human MR1, β2m, TRAV1–2–TRAJ33 and TRBV6-1 were expressed for 4 h in BL21 Escherichia coli after induction with 1 m M isopropyl β-D-1-thiogalactopyranoside. E. coli were pelleted and resuspended in a buffer containing 50 mM Tris, 25% (w/v) sucrose, 1 mM EDTA and 10 mM DTT pH 8.0. Inclusion-body protein was then extracted by lysis of bacteria in a buffer containing 50 mM Tris pH 8.0, 1% (w/v) Triton X-100, 1% (w/v) sodium deoxycholate, 100 mM NaCl, 10 mM DTT, 5 mM MgCl 2 and 1 mg DNaseI per litre of starting culture; the subsequent steps involved homogenization with a polytron homogenizer, centrifugation and washing inclusion-body protein sequentially, with (1) a buffer containing 50 mM Tris pH 8.0, 0.5% Triton X-100, 100 mM NaCl, 1 mM EDTA and 1 mM DTT, and (2) a buffer containing 50 mM Tris pH 8.0, 1 mM EDTA and 1 mM DTT. Inclusion-body protein was then resuspended in a buffer containing 20 mM Tris pH 8.0, 8 M urea, 0.5 mM EDTA and 1 mM DTT, and after centrifugation the supernatant containing solubilized, denatured inclusion-body protein was collected and stored at −80 °C. Refolding of MR1 and MAIT TCR The method for refolding and purifying the MR1-β2m–ligand complex is based on a similar methodology to that used for the classical MHC heavy-chain-β2m–peptide complex described in Kjer-Nielsen et al. [16] and Garboczi et al. [33] The refolded MR1-β2m–ligand complex was then purified by sequential DEAE (GE Healthcare) anion exchange, S75 16/60 (GE Healthcare) gel filtration and MonoQ (GE Healthcare) anion exchange chromatography. The TRAV1–2–TRAJ33–TRBV6-1 MAIT TCR was expressed, refolded and purified essentially as previously described [27] . Both the MR1-β2m–ligand and MAIT TCR were concentrated to 6 mg ml −1 and mixed in a ratio of 1:1 prior to crystallization. Structure determination Crystals of MAIT TCR–MR1-6-FP and MAIT TCR–MR1–RL-6-Me-7-OH complexes diffracted to 2 Å or better and belong to the space group C2 , with two molecules within the asymmetric unit. The data were processed using Mosflm version 7.0.5 (ref. 34 ) and scaled using SCALA from the CCP4 Suite [35] . The data for MAIT TCR–MR1–6-FP were solved by the molecular replacement method using PHASER in CCP4, with MR1 (PDB code 4GUP ) without the ligand and ELS4 TCR (PDB code 2NX5 ) without the loop region as a search model. The data for MAIT TCR–MR1–RL-6-Me-7-OH complex were solved using MAIT TCR–MR1–6-FP, without the ligand as a model. To prevent model bias, the R free set of the MAIT TCR–MR1–6-FP data was used in the experimental intensities scaling using SCALA as well as the implementation of the simulated annealing protocol in Phenix [36] . RL-6-Me-7-OH was modelled using the Dundee PRODRG2 server [37] . Both structures were refined using BUSTER 2.10 (ref. 38 ). Model building was carried out using COOT. The quality of the structure was validated at the Research Collaboratory for Structural Bioinformatics Protein Data Bank Data Validation and Deposition Services. All molecular graphics representations were created using PyMOL [39] . Surface area calculations were carried out using Areaimol within the CCP4 suite [35] . See Table 1 for data collection and refinement statistics. Surface plasmon resonance All surface plasmon resonance (SPR) experiments were conducted at 25 °C on a BIAcore 3000 instrument using HBS buffer (10 mM HEPES-HCl (pH 7.4), 150 mM NaCl). The biotinylated-MR1–Ag complexes were immobilized to an SA-Chip (GE) with a surface density of approximately 2,000 RU. Various concentrations of 6-1 MAIT TCR or MAIT TCR Y95F TCR (1.17–300 μM) were injected over the captured-MR1–Ag at 10 μl min −1 . The final response was calculated by subtracting the response of the blank flow cell alone from the MAIT TCR–MR1–Ag complex. The equilibrium data were analysed using GraphPad Prism. Assays of Jurkat cells transduced with MAIT TCR Jurkat cells transduced with a MAIT TCR comprising the TRAV1–2–TRAJ33 invariant α-chain and the TRBV6-1, TRBV6-4 or TRBV20 β-chains were tested for activation by co-incubation with ribityl lumazine compounds and C1R antigen-presenting cells expressing MR1. For inhibition experiments, 6-FP or a control pterin 6,7-dimethylpterin was added to C1R.MR1 cells (10 5 ) 30 min before the addition of activating ribityl lumazine compounds RL-6-Me-7-OH and rRL-6-CH 2 OH, after which Jurkat.MAIT cells (10 5 ) were added for 16 h. Cells were subsequently stained with PE-conjugated anti-CD3 and APC-conjugated anti-CD69 antibodies before analysis by flow cytometry. Activation of Jurkat.MAIT cells was measured by an increase in surface CD69 expression. Author Information : The atomic coordinates and structure factors for the TCR–MR1–Ag complexes were deposited in the Protein Data Bank (PDB codes 4L4V and 4L4T ). How to cite this article: Patel, O. et al. Recognition of vitamin B metabolites by mucosal-associated invariant T cells. Nat. Commun. 4:2142 doi: 10.1038/ncomms3142 (2013).